Towards hybrid superlattices in graphene The controllable and reversible modification of graphene by chemical functionalization can modulate its optical and electronic properties. Here we demonstrate the controlled patterning of graphane/graphene superlattices within a single sheet of graphene. By exchanging the sp 3 C–H bonds in graphane with sp 3 C–C bonds through functionalization, sophisticated multifunctional superlattices can be fabricated on both the macroscopic and microscopic scales. These patterns are visualized using fluorescence quenching microscopy techniques and confirmed using Raman spectroscopy. By tuning the extent of hydrogenation, the density of the sp 3 C functional groups on graphene's basal plane can be controlled from 0.4% to 3.5% with this two-step method. Using such a technique, which allows for both spatial and density control of the functional groups, a route to multifunctional electrical circuits and chemical sensors with specifically patterned recognition sites might be realized across a single graphene sheet, facilitating the development of graphene-based devices. Graphene has emerged as a remarkable material for diverse optoelectronics applications [1] , [2] , [3] , [4] , [5] , [6] owing to the large-scale synthetic routes to produce it in monolayer form, its extraordinary carrier mobility and conductivity, and its versatility for band structure engineering [1] , [7] , [8] , [9] , [10] , [11] , [12] , [13] , [14] , [15] , [16] . Controllably tailoring graphene's electronic structure with selective synthetic methods could better shape this two-dimensional semi-metal material for use in different applications. It is known that physisorption of chemical species on graphene can temporarily alter its electrical properties; however, adsorbates are too volatile for long-term usage [17] . With stronger binding energy and electronic coupling, covalent functionalization can permanently change the electronic structure of graphene. Hydrogenation is one straightforward route to render graphene, which has a bandgap of zero, into a wide-gap semiconductor, and recent studies have indicated that this method is controllable and reversible [1] , [2] . However, hydrogenation produces a single type of functional group, a sp 3 C–H bond, which may prevent the material from being useful in more complicated applications. To convert the proton into more diverse chemical substituents, an extra chemical step, functionalization using a diazonium salt reaction, is demonstrated here. Reaction of diazonium salts with mechanically cleaved graphene was found to be selective to the edges and defects rather than the basal plane [18] , [19] . However, for electronic applications of graphene, there is a need for more uniformity in grafting functionality to the surface. Here using the hydrogenated graphene as the activated precursor, C–H bonds are effectively exchanged with C–C bonds through diazonium salt functionalization, which controllably endows this material with a new spectrum of chemical and electrical properties. Furthermore, superlattices formed with built-in multifunctional regions in desired templates could yield characteristics necessary for the development of applications in, for example, chemical sensors, thermoelectrics and metamaterials [3] , [6] , [20] . In many cases, to produce materials relevant for these applications requires controlled attachment of complex molecules into patterns [21] . Alternatively, the ability to take a single template, such as graphene, and use existing processes such as lithographic patterning to create such structures on a molecular level, facilitates a route towards the rapid development of such desired architectures. The ability to produce large-scale graphene transferable to varied host surfaces also makes graphene an excellent template for the development of well-established top-down patterning approaches for device fabrication. Recent theoretical studies have emphasized the viability of this route for making quantum dots from patterned interfaces of hydrogenated and pristine graphene [22] , and we extend this idea to large-scale patterning of multifunctional domains on graphene. 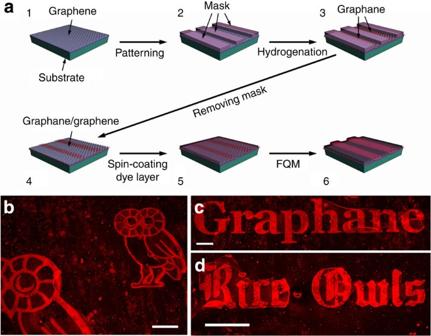Figure 1: Graphane/graphene superlattices fabrication and imaging. (a) Schematic illustration to fabricating the graphane/graphene superlattices and subsequent fluorescence quenching microscopy (FQM) imaging. (btod) FQM imaging of the graphene with different graphane/graphene patterns. The scale bars in b to d are 200 μm. Fabrication of the superlattices in graphene The typical process to pattern hydrogenated graphene domains and the subsequent imaging using fluorescence quenching microscopy (FQM) is illustrated in Figure 1a . First, large-area graphene, grown from Cu substrates by chemical vapour deposition or solid carbon methods, were transferred to an insulating substrate such as quartz or SiO 2 /Si, using the PMMA protection procedure as described elsewhere [11] , [12] . Following this, conventional photolithography was employed with a photoresist mask to define patterns atop the graphene films. Next, the exposed area of graphene was hydrogenated, using atomic hydrogen generated by a tungsten hot filament at low H 2 pressure (10 to 20 Torr). The sample takes 2 h to be hydrogenated thoroughly at ~10 °C (ref. 2 ). This procedure was found to be effective for controlled hydrogenation, minimizing graphene etching that originates at defects or edges [23] . Finally, the photoresist mask was removed to yield a conductive graphene sheet patterned with domains of insulating graphane-containing regions. Figure 1: Graphane/graphene superlattices fabrication and imaging. ( a ) Schematic illustration to fabricating the graphane/graphene superlattices and subsequent fluorescence quenching microscopy (FQM) imaging. ( b to d ) FQM imaging of the graphene with different graphane/graphene patterns. The scale bars in b to d are 200 μm. Full size image Imaging the superlattices in graphene Although the fabrication of the graphane/graphene superlattices, as we demonstrate here, was largely reliant on conventional techniques, the challenge is determining a straightforward and rapid method for imaging the product of the process, namely the substructure of the graphane/graphene hybrid material. Therefore, the FQM technique [4] , discovered by Kim et al ., was used to image the existing hybrid patterns. According to the excited-state energy transfer mechanism, graphene may serve as an acceptor to quench the fluorescence of a thin spin-coated dye layer (0.02% rhodamine B mixed with 5% PMMA in acetone) [4] . Because graphene and its functionalized form are different in their conjugation, the differential quenching ability of the hybrid graphane/graphene pattern can be readily observed using FQM [4] . Using the technique illustrated in Figure 1a , graphane/graphene patterns have been made with photolithography and hydrogenation, and then imaged with FQM as shown in Figure 1b–d . In the photos, all of the dark areas are pristine graphene, which more efficiently quenches the fluorescence of the thin top dye layer. The bright areas are graphane; its fluorescence quenching ability is much weaker than in graphene because of the loss of conjugation in the former. This verifies that the formation of insulating domains on a conductive graphene sheet can be readily achieved. The bright spots or bands in the FQM images come from the aggregation and non-uniform coating of the dye layers, arising in part from the folds induced during transfer of the original graphene film. In all cases conventional photolithography was used, which is only capable of accuracy down to length scales of ~1 μm in our laboratory ( Supplementary Fig. S1 ). However, well-defined structures that can be achieved using more advanced lithographic techniques can extend this technique to finer patterning [24] . 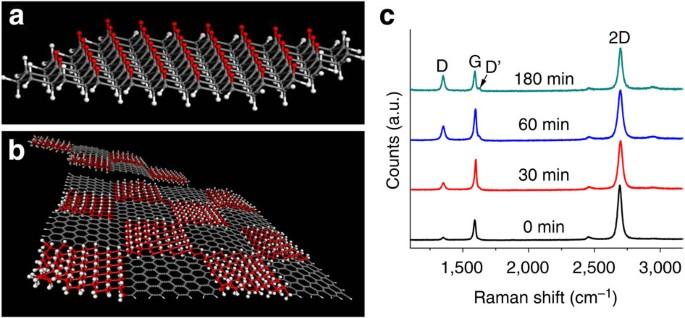Figure 2: Molecular models of graphane and graphane/graphene superlattices and corresponding Raman spectra of experimental products. (a) Fully hydrogenated graphene structure. (b) Graphane/graphene superlattices structures. (c) Raman spectra of graphene and graphane with extended hydrogenation time. The D peak increases as the hydrogenation time increases from 0 min (bottom) to 180 min (top). Towards hybrid superlattices in graphene Typical atomic models of graphane and graphane/graphene superlattices are shown in Figure 2a,b . Although, in our cases, full hydrogenation is not achieved because of the substrate hindering effect, the hydrogenated section has more sp 3 carbon characteristics than does the pristine section, as seen by the pronounced D peak in the Raman spectrum. The Raman spectra displayed in Figure 2c correspond well with those reported for single-layer graphene before and after hydrogenation [2] . With extended hydrogenation time, more sp 3 C characteristics or higher D peaks were observed. In Raman spectra of pristine monolayer graphene, the D peak (1,350 cm −1 ) is much lower than the G peak (1,580 cm −1 ), and the 2D peak (2,685 cm −1 ) is about 4 times more intense than the G peak. After 180 min of hydrogenation, the D peak is almost as high as the G peak. An extra D' peak (1,620 cm −1 ) is detected on the shoulder of the G peak, and the 2D peak is suppressed because of the chemical functionalization. The D peak intensity was also recorded as a 2-dimensional map to confirm the formation of a graphene/graphane patterns in Supplementary Figure S2 . However, compared with FQM that only takes a few seconds to image a large area of the sample, Raman mapping is relatively time-consuming (7 h for 50 μm×50 μm area in Supplementary Fig. S2 ) with a resolution limited by the laser spot size of the Raman instrument. Four-probe electrical measurements before and after the hydrogenation demonstrate a gradual transformation from semi-metallic graphene to near-insulating graphane-like material. After annealing at 520 °C for 30 min under high vacuum (10 −6 –10 −7 Torr), the graphane is partially converted back to graphene based on the partial recovery of its conductivity ( Supplementary Fig. S3 ). This provides further evidence that insulating graphane domains formed from a conductive graphene template [2] . Figure 2: Molecular models of graphane and graphane/graphene superlattices and corresponding Raman spectra of experimental products. ( a ) Fully hydrogenated graphene structure. ( b ) Graphane/graphene superlattices structures. ( c ) Raman spectra of graphene and graphane with extended hydrogenation time. The D peak increases as the hydrogenation time increases from 0 min (bottom) to 180 min (top). Full size image With this graphane/graphene superlattice in hand, the material can be additionally functionalized using diazonium salts. The diazonium salt reaction with the graphane/graphene intermediate is most likely to go through a free radical mechanism, as had been proposed for the diazonium functionalization of a hydrogen-passivated Si surface [25] . 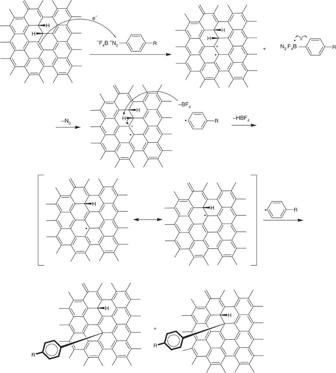Figure 3: Diazonium reaction with hydrogenated graphene. A proposed mechanism of spontaneous diazonium activation by a hydrogenated graphene surface. Only two regioisomers are shown in the final product, though others are possible. As shown in Figure 3 , in this case, we propose a spontaneous electron transfer from the surface of the graphane/graphene substrate to the diazonium salt, generating an aryl radical on loss of N 2 and a graphane/graphene radical cation. A proton is eliminated from the graphane/graphene to form HBF 4 and a graphane/graphene radical. Within a common solvent shell, the free aryl radicals attack the surface near the sp 3 C–H bond sites to form the new covalent sp 3 C–C bonds. Figure 3: Diazonium reaction with hydrogenated graphene. A proposed mechanism of spontaneous diazonium activation by a hydrogenated graphene surface. Only two regioisomers are shown in the final product, though others are possible. Full size image Thermodynamically, pristine graphene is inert to many organic reactions except at structurally reactive spots with relatively high chemical potential, which make these latter sites more reactive. For example, the edges, strain sites (ripples) and the Stone-Wale defects are more reactive than the crystalline basal planes of graphene, based on experimental and theoretical studies [19] , [26] , [27] . Nevertheless, hydrogenation functionalizes the basal plane of graphene in a controllable, uniform and reversible manner. Here we show that hydrogenation also activates the basal plane towards diazonium functionalization. Similar to aryl radicals in the diazonium reaction, the atomic H works as a free radical (H•). This H-radical generated by the hot tungsten filament overcomes the high-energy barrier to break the sp 2 bond in graphene and it, thereby, forms a new sp 3 bond. Supplementary Figure S4 displays the reaction energy scheme for both the direct diazonium reaction (addition reaction, sp 2 bond to sp 3 bond) and the diazonium reaction after hydrogenation (substitution reaction, sp 3 bond to sp 3 bond). 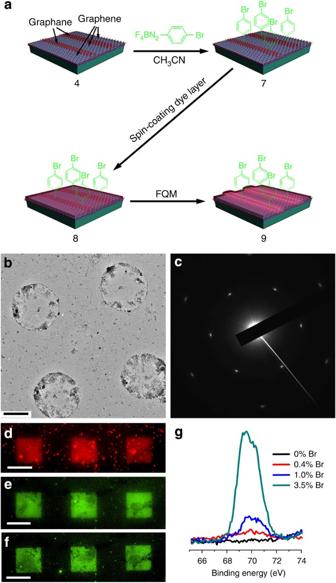Figure 4: Controllable exchange of sp3C–H bonds with sp3C–C bonds using 4-bromophenyldiazonium tetrafluoroborate. (a) Schematic illustration of the fabrication of sp3C–C exchanged superlattices and subsequent FQM imaging. (b) TEM image of diazonium functionalized graphene film covering a TEM grid with four suspended areas shown. The scale bar in b is 0.5 μm. (c) Selected area electron diffraction (SAED) pattern of diazonium functionalized graphene. (dtof) FQM images of diazonium functionalized graphene superlattices. The dye molecules used in FQM are rhodamine B in (d), FITC in (e) and fluorescein sodium in (f). The scale bars indtofare 50 μm. (g) XPS of samples containing different percentages of 4-bromophenylene functionality by tuning the hydrogenation process. The bromine content could be controlled from 0 to 3.5%. The diazonium reaction and FQM experiment to image the hybrid superlattices were performed as shown in Figure 4a . Figure 4: Controllable exchange of sp 3 C–H bonds with sp 3 C–C bonds using 4-bromophenyldiazonium tetrafluoroborate. ( a ) Schematic illustration of the fabrication of sp 3 C–C exchanged superlattices and subsequent FQM imaging. ( b ) TEM image of diazonium functionalized graphene film covering a TEM grid with four suspended areas shown. The scale bar in b is 0.5 μm. ( c ) Selected area electron diffraction (SAED) pattern of diazonium functionalized graphene. ( d to f ) FQM images of diazonium functionalized graphene superlattices. The dye molecules used in FQM are rhodamine B in ( d ), FITC in ( e ) and fluorescein sodium in ( f ). The scale bars in d to f are 50 μm. ( g ) XPS of samples containing different percentages of 4-bromophenylene functionality by tuning the hydrogenation process. The bromine content could be controlled from 0 to 3.5%. Full size image The diazonium functionalized graphene film was lifted off from a SiO 2 /Si wafer and transferred onto a c-flat transmission electron microscope (TEM) grid (Protochips) with the PMMA protection method [12] . The etchant used here is buffered oxide etchant (J.T. Baker, Buffered Oxide Etch 6:1). In Figure 4b,c , the TEM image and selected area electron diffraction pattern prove that the graphene sample is maintained after the chemical process of hydrogenation and diazonium reaction. FQM was used to image the same diazonium-functionalized graphene superlattices with different dye molecules, such as rhodamine B, fluorescein isothiocyanate (FITC), and fluorescein sodium in Figure 4d–f , respectively. The diazonium functionality introduced was determined by analysis of the bromine content of the functionalized product using X-ray photoelectron spectroscopy (XPS); the Br content was due to the 4-bromophenyldiazonium tetrafluoroborate used in the functionalization. As shown in Figure 4g , under the same reaction conditions, pristine graphene has only 0.4% bromine content after functionalization with the diazonium salt, whereas graphane has bromine content >1%. The more graphane that is present in the sample, the more bromophenyl-functionalization that is introduced. The sample with the most graphane had a bromine content of 3.5%, which is approximately one new sp 3 C–C bond in every 21.5 C atoms in the graphane domains. With this two-step functionalization method, graphene's basal surface can be controllably grafted with Br content up to 3.5%, with a lithographically defined spacial resolution. Furthermore, to visualize the patterns, we used FQM, which, when combined with Raman spectroscopy, provides the necessary analytical tools to characterize the heterostructures. The two-step controlled covalent functionalization process described here permits modulation of the electronic properties of graphene's basal planes and could hold promise for specifically patterned optoelectronic and sensor devices based on this exciting new material. Graphane/graphene superlattices fabrication Graphene films were grown on 25-μm thick Cu foils (99.8%, Alfa Aesar, item No. 13382) and transferred onto various substrates, such as glass, quartz, and 100 nm SiO 2 /Si, according to the methods reported [1] , [2] . Graphene patterns were fabricated using a photoresist (Microposit S1813) mask in a standard photolithography process or a PMMA mask in an e-beam lithography process. Hydrogenation was performed in a vacuum system equipped with a hot tungsten filament (diameter=0.25 mm, 99.95%, Alfa Aesar) that splits the H 2 gas into H atoms. Before the hydrogenation, the graphene samples (or graphene patterns) were heated in vacuum (10 −6 Torr) at 400 °C (200 °C with polymer-defined patterns) for 15 min to remove physisorbed polymers and other contaminants that might block the hydrogenation of the graphene surface. 50 sccm H 2 was then introduced into the system and the pressure was controlled at ~10 Torr using a valve connected to the vacuum pump. The filament current was slowly increased to ~13 A and the total power was maintained at ~60~65 W. The graphene samples were placed ~2 cm from hot filament for various times (15 min, 30 min, 1 h, 2 h or 3 h) to produce different levels of hydrogenation. The FQM pattern samples were made from the superlattices that had been hydrogenated for 2 h. After the hydrogenation, the polymer masks were removed by rinsing with 10 ml acetone 3×. FQM imaging of the superlattices A thin layer of dye (0.02 wt% Rhodamine B, FITC or fluorescein sodium, mixed with 5 wt% PMMA acetone solution) was deposited onto the superlattice sample surfaces by spin-coating at 5,000 rpm for 1 min (Headway Research). The samples were imaged under a fluorescence microscope (Zeiss Axioplan 2 imaging optical microscope). It was equipped with a Mercury Arc lamp (HBO 100 W) and in combination with a set of filters, coordinates the excitation and emission wavelengths corresponding to a particular fluorophore. In this work, Texas of Red (Ex: 555, 595/Em: 615 nm) and Cy3 (Ex: 514, 554/Em: 566, 615 nm) channels were used for rhodamine B, and FITC (Ex: 493/Em: 517 nm) channel was used for FITC and fluorescein sodium. Images were recorded and processed at room temperature using a Photometrics Cool Snap HQ camera and MetaMorph software. The objectives used were ×10, ×20, and ×40 in air; ×63 and ×100 in oil. The diazonium functionalized graphane/graphene superlattices have the same contrast as the unfunctionalized precursors, namely the graphane/graphene superlattices. Diazonium functionalization of the hydrogenated graphene In the diazonium functionalization experiments, the substrates (graphene hydrogenated for varied times of 0, 15, 30, 60, 120 to 180 min) were placed in a N 2 -purged, freshly prepared mg ml −1 diazonium salt solution (4-bromobenzenediazonium tetrafluoroborate in CH 3 CN) in the dark at room temperature for 20 h. The reactions could also be performed under UV light (254 nm) in 2 h. After the diazonium reaction, the samples were rinsed in CH 3 CN 3× to thoroughly remove any physisorbed diazonium salt residue and they were then dried using a flow of N 2 before further characterization. Spectroscopic characterizations The Raman spectroscopy and mapping was performed on graphane/graphene superlattice films on quartz substrates using 514-nm laser excitation at room temperature with a Renishaw Raman RE02 microscope. XPS was performed using a PHI Quantera SXM scanning X-ray microprobe with 45° takeoff angle and a100-μm beam size. How to cite this article: Sun, Z. et al . Towards hybrid superlattices in graphene. Nat. Commun. x:x doi: 10.1038/ncomms1577 (2011).